Surpassing the single-atom catalytic activity limit through paired Pt-O-Pt ensemble built from isolated Pt1atoms Despite the maximized metal dispersion offered by single-atom catalysts, further improvement of intrinsic activity can be hindered by the lack of neighboring metal atoms in these systems. Here we report the use of isolated Pt 1 atoms on ceria as “seeds” to develop a Pt-O-Pt ensemble, which is well-represented by a Pt 8 O 14 model cluster that retains 100% metal dispersion. The Pt atom in the ensemble is 100–1000 times more active than their single-atom Pt 1 /CeO 2 parent in catalyzing the low-temperature CO oxidation under oxygen-rich conditions. Rather than the Pt-O-Ce interfacial catalysis, the stable catalytic unit is the Pt-O-Pt site itself without participation of oxygen from the 10–30 nm-size ceria support. Similar Pt-O-Pt sites can be built on various ceria and even alumina, distinguishable by facile activation of oxygen through the paired Pt-O-Pt atoms. Extending this design to other reaction systems is a likely outcome of the findings reported here. An ideal supported metal catalyst will simultaneously maximize dispersion of the metal and display optimal intrinsic activity per metal atom. Recently, advanced techniques for synthesizing many heterogeneous catalysts as single atoms have addressed the former issue. Single-atom catalysis dramatically reduces the usage requirements of expensive and rare metals by stabilizing the supported metal atoms in a fully dispersed state as isolated bonded species that serve as active sites [1] , [2] , [3] , [4] , [5] , [6] . A general question regarding single-atom metal catalysts, despite the nearly 100% material efficiency of the supported metals, is whether a catalytic center designed in the form of one metal atom substituted or anchored on a support represents the optimal structure to deliver the highest intrinsic catalytic activity. Previous work answered this question for platinum and gold catalysts for the water–gas shift reaction, where the optimal catalytic center is the single-atom Pt 1 (or Au 1 )-O(OH) x species on a variety of catalyst supports [4] , [5] , [6] . Nonetheless, for other important reactions such as the low-temperature CO oxidation, these configurations as isolated atomic active sites may lack neighboring metal centers and the reactivities associated with the latter. This fundamental question remains unanswered and industrial needs for more active catalysts await. The catalytic oxidation of CO to CO 2 involves classic molecular rearrangements with oxygen intermediates that make it an attractive probe reaction in catalytic systems to gain better mechanistic understanding, such as the identity of metal catalytic centers and the importance of metal–support interaction. The low-temperature CO oxidation is also important in the purification of vehicle emissions. To meet latest fuel-efficient engine designs and to reduce vehicle exhaust emissions, platinum group metals (PGMs) dispersed on ceria supports are needed to be much more active in eliminating CO emissions below 150 °C during the engine cold start [7] . A group of Pt single-atom catalysts using CeO 2 [8] , [9] , Al 2 O 3 [10] , [11] , and KLTL zeolite [12] supports were developed and probed for CO oxidation. Compared with the conventional Pt nanoparticles where most of the metal atoms are buried inside the particle bulk without catalyzing the surface reaction, these single-atom catalysts certainly facilitate the full utilization of scarce platinum metal [4] , [5] , [6] , [8] , [9] . However, the properties of the Pt 1 may be suboptimal for certain reactions. 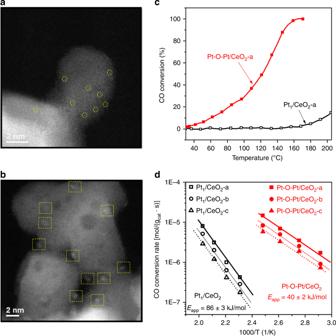Fig. 1 Direct measurements of the Pt1/CeO2and Pt-O-Pt/CeO2catalysts.a,bAberration-corrected high-angle annular dark-field scanning transmission electron microscopy (HAADF-STEM) images for the Pt1/CeO2-a and Pt-O-Pt/CeO2-a catalysts (shown images were recorded at ×10 M and ×6 M original magnifications, respectively). Yellow circles and squares are used to highlight the single-atom Pt1and the Pt-O-Pt ensemble, respectively.cCO oxidation light-off performance ([CO] = 1000 ppm, [O2] = 5%, balanced with N2at a contact time of 2,400,000 mL/gcat//h).dArrhenius-type plot of CO oxidation rates at different temperatures with apparent activation energies (Eapp) shown Indeed, a closer examination of the activity per Pt atom shows that such Pt 1 catalysts are often similar to (or even worse than [3] ) the conventional Pt nanoparticles and clusters under comparable reaction conditions and catalyst formulations (Supplementary Table 1 ). In the context of oxygen-rich reaction conditions (oxygen in excess to fully oxidize all the reductants), which reflects the implementation of emerging fuel saving technologies such as lean-burn engines, hybrid powertrains, and dynamic fuel management, the known benefit of creating oxygen vacancies on ceria surfaces to promote CO oxidation under near stoichiometric oxygen concentrations [13] , [14] , [15] cannot be sustained because the surface oxygen vacancies associated with Ce(III) heal in seconds [16] , [17] . Consequently, the natural question arises whether a properly paired multi-atom catalytic site (ensemble of the single-atom M 1 -O x species) will increase the catalytic performance over Pt 1 /CeO 2 under oxygen-rich conditions, and how we can build such a site with an appreciable loading amount on a given support surface. In this work, by extending the concept of isolated atoms to the paired ensembles, we show that the paired Pt-O-Pt catalytic units can achieve higher activity through an oxygen migration mechanism. Here we report a general approach—reassembling isolated Pt 1 atoms as the precursor to create a one-layer multi-atom oxo site (Pt-O-Pt) while keeping ~100% Pt utilization. We use a variety of experimental and computational techniques (grand canonical Monte Carlo (GCMC) simulations combined with density functional theory (DFT) calculations (GCMC-DFT) [18] to elucidate the catalyst active site structure and the CO oxidation reaction mechanism that is responsible for the dramatically enhanced reactivity of this multi-atom oxo site. The Pt-O-Pt ensemble is shown to be the base unit in the high-performance catalyst, where the well-known Pt-CeO 2 metal–support interfacial catalysis no longer ranks as the favorable reaction path for this highly active low-temperature CO oxidation catalyst under oxygen-rich reaction conditions. Dramatic change of catalytic performance We began this work by synthesizing a variety of single-atom Pt 1 /CeO 2 to serve as the baseline for catalytic performance. Next, the isolated Pt atoms in the Pt 1 /CeO 2 were used as seeds to generate a much more active Pt site through a facile activation treatment, where a mild H 2 reduction was followed with a CO plus O 2 treatment to trigger the restructuring of the platinum (see optimization of the activation treatment and the stable, high reaction rates in Supplementary Figs. 1 – 3 . The optimized samples are labeled as Pt-O-Pt/CeO 2 , see Table 1 ). The potential alternative activity contributors, such as creating persistent oxygen vacancies and additional –OH species on the catalyst surface during the activation treatment, have been excluded (Supplementary Figs. 4 and 5 ). Table 1 Key metrics of the Pt 1 /CeO 2 and the Pt-O-Pt/CeO 2 catalysts Full size table Aberration-corrected high-angle annular dark-field scanning transmission electron microscopy (HAADF-STEM) images show that the single Pt atoms are the majority species in the various Pt 1 /CeO 2 samples prepared in this work (see Fig. 1a and Supplementary Figs. 6 – 8 for Pt 1 /CeO 2 -a, Pt 1 /CeO 2 -b, and Pt 1 /CeO 2 -c samples), where Pt loadings of 0.27, 0.16, and 0.11 wt.% and ceria supports with diverse amounts of reducible oxygen species were used (Supplementary Figs. 9 and 10 ). A few pseudo-clusters of platinum might be found in these single-atom catalyst samples, where these pseudo-clusters are composed of several nearby single-atom Pt 1 species embedded in the cerium columns. In the activated catalysts, namely the Pt-O-Pt/CeO 2 samples, the Pt atoms are fully transformed into another structure with a narrow size distribution of 1 ± 0.1 nm on the ceria surface (see Fig. 1b and Supplementary Figs. 11 – 13 for Pt-O-Pt/CeO 2 -a, Pt-O-Pt/CeO 2 -b, and Pt-O-Pt/CeO 2 -c samples). We measure the Pt dispersion of Pt-O-Pt/CeO 2 samples to be nearly 100% (Table 1 ). Additional STEM images and discussion of the representative Pt 1 /CeO 2 -a and Pt-O-Pt/CeO 2 -a samples can be found in Supplementary Figs. 14 and 15 and their accompanying text. None of the crystal patterns for platinum metal or oxides were detected in the Pt-O-Pt/CeO 2 catalysts by either STEM imaging or X-ray diffraction (Fig. 1b and Supplementary Figs. 11 – 13 , 15 , and 16 ), meaning that only the highly dispersed platinum species reside on the predominant CeO 2 (111) surfaces (Supplementary Fig. 17 ) with ceria nanoparticle sizes of 10–30 nm. There are some rounded edges, steps, and kinks on these rather typical industrial CeO 2 support particles, but no clear evidence of these locations as the preferred anchoring sites for the platinum species is found (Supplementary Fig. 18 ). Therefore, we selected CeO 2 (111) to model the stable geometry and CO oxidation reaction path for Pt 1 /CeO 2 and Pt-O-Pt/CeO 2 . Fig. 1 Direct measurements of the Pt 1 /CeO 2 and Pt-O-Pt/CeO 2 catalysts. a , b Aberration-corrected high-angle annular dark-field scanning transmission electron microscopy (HAADF-STEM) images for the Pt 1 /CeO 2 -a and Pt-O-Pt/CeO 2 -a catalysts (shown images were recorded at ×10 M and ×6 M original magnifications, respectively). Yellow circles and squares are used to highlight the single-atom Pt 1 and the Pt-O-Pt ensemble, respectively. c CO oxidation light-off performance ([CO] = 1000 ppm, [O 2 ] = 5%, balanced with N 2 at a contact time of 2,400,000 mL/g cat //h). d Arrhenius-type plot of CO oxidation rates at different temperatures with apparent activation energies ( E app ) shown Full size image Despite the apparently low conversion values on the Pt 1 /CeO 2 catalysts (Fig. 1c and Supplementary Fig. 19 ), which are due to the high gas flow rate compared to catalyst weight, the absolute (or intrinsic) activities of our single-atom Pt for low-temperature CO oxidation per Pt site (turnover frequencies, TOFs) are within the same order of magnitude as the activities reported recently for other single-atom Pt catalysts [8] , [9] , [10] , [11] , [12] , [19] , [20] , [21] , [22] , [23] , [24] , particularly when reducible oxide supports such as titania and ceria were used (Supplementary Table 1 ). Under the same reaction conditions, however, the Pt-O-Pt/CeO 2 catalysts have 2–3 orders of magnitude higher intrinsic activity than their Pt 1 /CeO 2 counterparts from 80 to 150 °C. The reaction rates on the Pt 1 /CeO 2 -a catalyst are 1.7 × 10 –9 and 2.2 × 10 –7 mol CO 2 /(g cat ·s) at 80 and 150 °C, respectively. In contrast, at the same total platinum loading, the reaction rates on the Pt-O-Pt/CeO 2 -a catalyst are 2.6 × 10 −6 and 2.5 × 10 −5 mol/(g cat ·s) at 80 and 150 °C. Kinetic measurements (Fig. 1d ) further reveal that the Pt-O-Pt/CeO 2 and Pt 1 /CeO 2 catalysts are also distinguishable from differences between their catalytic centers and reaction mechanisms. Specifically, the CO oxidation reaction catalyzed by the Pt-O-Pt/CeO 2 catalysts has a smaller measured apparent activation energy ( E app = 40 ± 2 kJ/mol) compared with the Pt 1 /CeO 2 catalysts ( E app = 86 ± 3 kJ/mol). In agreement with earlier studies on metal nanoparticle catalysts [25] , [26] , recent reports have confirmed the benefit of H 2 O and its dissociated –OH species for promoting CO oxidation on Pt 1 /CeO 2 catalysts [9] , [19] . In our case, an activity improvement for both Pt-O-Pt/CeO 2 and Pt 1 /CeO 2 catalysts is observed after adding 3% H 2 O into the CO oxidation feed stream (Supplementary Fig. 20 ), but the large activity gap between the Pt-O-Pt/CeO 2 and Pt 1 /CeO 2 samples remained. This result proves that the beneficial H 2 O/–OH-rich environment [9] , [19] , [25] , [26] does not diminish the superior activity of the Pt-O-Pt/CeO 2 over its Pt 1 /CeO 2 counterpart. Despite the further complication of reaction routes due to the water-containing experiment, these data demonstrated that the relative activity of the Pt-O-Pt structure compared with Pt 1 /CeO 2 will not be negated even in the presence of water and –OH-enriched environment. The activated Pt-O-Pt/CeO 2 -a sample remains similarly active even after being hydrothermally aged at 750 °C for 20 h (Supplementary Fig. 20 ). Further evidence of the generalizability of this synthetic approach to effectively construct the active Pt-O-Pt catalytic center is shown on two types of commercial platinum–ceria catalysts (Supplementary Figs. 21 and 22 ). Atomic-level structural analyses Our DFT calculations identified the stable Pt structures for the Pt 1 /CeO 2 and Pt-O-Pt/CeO 2 catalysts. We find that the isolated Pt 1 atom prefers to substitute the Ce atom rather than anchor on the CeO 2 (111) surface (the dominant facet on which ~70% counts of the experimental Pt 1 and ~1 nm Pt-O-Pt species were anchored, Supplementary Fig. 17 ). This Pt 1 anchoring site was proposed in a prior experimental study [27] . The Pt 1 anchored on top of the CeO 2 (111) is thermodynamically unstable due to a highly unsaturated coordination environment (Supplementary Fig. 23a ). In the identified Pt 1 /CeO 2 structure (Fig. 2a and Supplementary Figs. 23b and 24 ), the Pt 1 substitutes the Ce atom on the ceria surface and is surrounded by up to six nearby oxygen atoms. In line with the recent findings from surface science and DFT calculations studies [28] , [29] , we noticed that four of the oxygen atoms prefer to bind directly to the Pt center to form a square-planar Pt 1 -O 4 structure, which is the starting structure of the Pt 1 /CeO 2 catalysts used here to model the CO oxidation reaction. Fig. 2 The density functional theory (DFT)-optimized Pt structures and the material characterization results. a , b DFT-optimized structure of representative single-atom Pt in the Pt 1 /CeO 2 sample and Pt 8 O 14 in the Pt-O-Pt/CeO 2 sample found by grand canonical Monte Carlo-DFT (GCMC-DFT). c Normalized Pt L 3 edge x-ray absorption near-edge structure (XANES) spectra and d Pt 4 f x-ray photoelectron spectroscopy (XPS) spectra of the Pt 1 /CeO 2 -a and the Pt-O-Pt/CeO 2 -a catalysts. e Fourier transform of extended X-ray absorption fine structure (EXAFS) spectra of Pt L 3 edge (phase corrected) for the Pt 1 /CeO 2 -a and Pt-O-Pt/CeO 2 -a catalysts. The first shell Pt-Pt coordination is not observed in the Pt 1 /CeO 2 and Pt-O-Pt/CeO 2 catalysts. The gray and red open circles are fitted curves for the Pt 1 /CeO 2 and Pt-O-Pt/CeO 2 catalysts, respectively. The PtO 2 standard is in the β-phase. f In situ diffuse reflectance infrared Fourier-transform spectroscopy (DRIFTS) under the CO oxidation conditions for the Pt 1 /CeO 2 -a and Pt-O-Pt/CeO 2 -a catalysts. DFT-predicted CO adsorption modes are shown inset for Pt 1 /CeO 2 − x and Pt 8 O 13 /CeO 2 . Color legend of atoms: Ce = beige; Pt = blue; C = gray; O (in CeO 2 and Pt 8 O 13 ) = red; O (in CO) = green Full size image Computationally intensive GCMC-DFT simulations were performed to search the structure and composition of Pt 8 /CeO 2 in the presence of oxygen ( \(p_{\mathrm{O}_{2}}\) = 0.05 atm) at 350 K, which is consistent with the experimental reaction conditions. The computationally tractable Pt 8 cluster was selected here because the experimental Pt-O-Pt/CeO 2 sample has a similar platinum diameter of ~1 nm on the CeO 2 (111) surfaces (Supplementary Fig. 25a ). When exposed to an oxygen atmosphere as in our reaction tests, the Pt 8 /CeO 2 rearranges into Pt 8 O 14 (~0.92 nm), which contains solely Pt-O-Pt as the catalytic base unit and is only one layer thick (Fig. 2b and Supplementary Fig. 26b ). Our GCMC simulation is similar with the experimental activation procedure in that the reduced Pt x clusters, formed by assembling Pt 1 species under the first step of H 2 treatment, can be oxidized to the Pt-O-Pt ensemble by the introduction of an O 2 -rich environment. The Pt 8 O 14 cluster model identified by the GCMC algorithm is regarded as a representative structure of our experimental system, as in reality some experimental heterogeneity does exist. Nevertheless, as we show below it captures many of the salient features of this rather clean experimental catalytic system, as indicated by the overall agreement of experimental observations and computational predictions. Since our synthesis of the Pt 1 /CeO 2 and Pt-O-Pt/CeO 2 catalysts yields almost exclusively either single-atom Pt 1 species or the ~1 nm Pt-O-Pt structure on the different ceria supports, the representative Pt 8 O 14 structure predicted by GCMC-DFT can be vetted by our experimental analysis. The x-ray absorption near-edge structure (XANES) and the x-ray photoelectron spectroscopy (XPS) results (Fig. 2c–d and Supplementary Figs. 26 and 27 ) confirm the cationic nature of the Pt atoms in both groups of catalysts. The Pt chemical valence in Pt 1 /CeO 2 is Pt(IV) and is slightly more positive than the Pt in the Pt-O-Pt/CeO 2 samples. 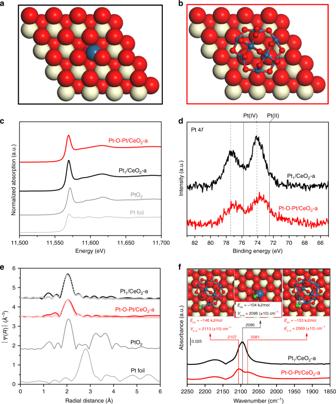Fig. 2 The density functional theory (DFT)-optimized Pt structures and the material characterization results.a,bDFT-optimized structure of representative single-atom Pt in the Pt1/CeO2sample and Pt8O14in the Pt-O-Pt/CeO2sample found by grand canonical Monte Carlo-DFT (GCMC-DFT).cNormalized Pt L3edge x-ray absorption near-edge structure (XANES) spectra anddPt 4fx-ray photoelectron spectroscopy (XPS) spectra of the Pt1/CeO2-a and the Pt-O-Pt/CeO2-a catalysts.eFourier transform of extended X-ray absorption fine structure (EXAFS) spectra of Pt L3edge (phase corrected) for the Pt1/CeO2-a and Pt-O-Pt/CeO2-a catalysts. The first shell Pt-Pt coordination is not observed in the Pt1/CeO2and Pt-O-Pt/CeO2catalysts. The gray and red open circles are fitted curves for the Pt1/CeO2and Pt-O-Pt/CeO2catalysts, respectively. The PtO2standard is in the β-phase.fIn situ diffuse reflectance infrared Fourier-transform spectroscopy (DRIFTS) under the CO oxidation conditions for the Pt1/CeO2-a and Pt-O-Pt/CeO2-a catalysts. DFT-predicted CO adsorption modes are shown inset for Pt1/CeO2 −xand Pt8O13/CeO2. Color legend of atoms: Ce = beige; Pt = blue; C = gray; O (in CeO2and Pt8O13) = red; O (in CO) = green Bader charge analysis of the predicted catalyst structures shows the same trend (Supplementary Table 2 ). Extended X-ray absorption fine structure (EXAFS) measurements (Fig. 2e , Supplementary Fig. 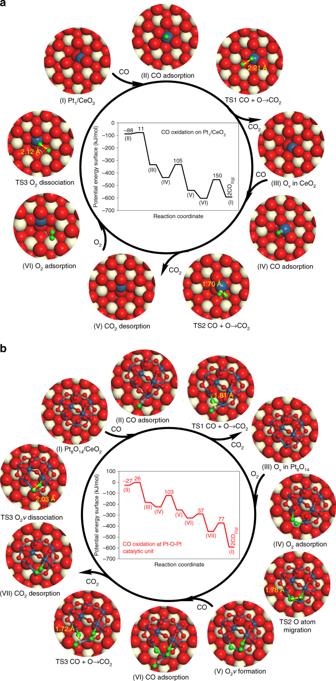Fig. 3 Potential energy diagrams and configurations for CO oxidation cycle. CO oxidation proceeds onathe Pt1/CeO2andbat the Pt-O-Pt catalytic unit in Pt8O14/CeO2. CO adsorption energies and reaction barriers are indicated in kJ/mol in the potential energy diagram. The bond distance between the two fragments at the transition state (TS) is given in angstrom (Å) in the configurations of CO oxidation. Beige, red, and blue spheres are Ce, O, and Pt atoms, respectively. The small gray and green spheres are C and O atoms involved in CO oxidation. Corresponding energetics are given in Supplementary Table4 28 , and Supplementary Table 3 ) show the typical exclusive Pt-O coordination environment (up to six nearby O atoms) for Pt 1 /CeO 2 . For the Pt-O-Pt/CeO 2 samples, unlike the prevalent three-dimensional platinum (oxide) clusters that possess more than one Pt layer and the resulting Pt-Pt coordination from EXAFS in a radial distance between 2.5 and 3.0 Å [30] , [31] , the Pt atoms of Pt-O-Pt/CeO 2 are only bridged by oxygen in its first shell coordination, making these Pt atoms share a high level of similarity to the isolated Pt 1 atom in terms of the Pt-O local structures (see XPS and XAS results in Fig. 2 , Supplementary Figs. 26 – 28 , and Supplementary Table 3 ). Consistent with the EXAFS measurements, the GCMC-predicted Pt 8 O 14 structure is composed of eight fully separated Pt cations, each bound to four nearby oxygen atoms with the average Pt-O distance of 1.99 Å. The lack of long-distance Pt-Pt and second shell Pt-O information for the Pt-O-Pt/CeO 2 catalysts at higher radial distances ( R > 3 Å) is the result of experimental signal dampening by the one-layer platinum structure, dilute platinum concentrations, and inherent signal attenuation in EXAFS analyses. These factors are discussed in the Supplementary Information accompanying Supplementary Fig. 29 . Diffuse reflectance infrared Fourier-transform spectroscopy (DRIFTS) studies under the CO oxidation conditions (Fig. 2f and Supplementary Fig. 30 ) reveal one dominant vibrational mode at 2095 cm −1 for the Pt 1 /CeO 2 samples, as reported in the literature [9] . A Pt 1 anchored on CeO 2 (111) can be ruled out because of its highly endothermic formation energy (Supplementary Fig. 23a ) and its strong CO adsorption ( E CO = −313 kJ/mol) with a calculated CO wavenumber of 2070 cm −1 , which is not observed in our DRIFTS measurement. The structure of Pt 1 substituted in the CeO 2 (111) surface is more stable and the calculated CO wavenumber of 2095 cm −1 on Pt 1 /CeO 2 − x (111) with one oxygen vacancy nearby is in line with our experimental measurement. The two sets of experimentally measured CO adsorption bands centered at 2107 and 2081 cm −1 for the Pt-O-Pt/CeO 2 samples correspond to CO chemisorption at the top and bridge sites of an undercoordinated Pt-O-Pt ensemble, according to our representative Pt 8 O 13 /CeO 2 (111) model system (identified after examination of all possible CO adsorption sites on Pt 8 O x ( x = 13−14) involved in the CO oxidation cycle). On Pt 8 O 13 /CeO 2 (111), CO chemisorption is −146 and −153 kJ/mol at the top and bridge site, respectively (Fig. 2f and Supplementary Figs. 30 and 31 ). Adsorbed CO can interchange between the bridge site and the top site. This evidence does not necessarily corroborate that these CO adsorption modes must belong to the reaction intermediates of the most energy-favored reaction pathways. Also, although the calculated frequencies of adsorbed CO on Pt 8 O 13 /CeO 2 have similar values compared with the experimental peak centers, we cannot exclude the other possible CO adsorption modes on any heterogeneous PtO x species in the Pt-O-Pt/CeO 2 catalyst. This limitation is also evidenced and discussed from the perspective of experimental DRIFTS results (Supplementary Fig. 30 ). We emphasize that the C-O vibrational frequency alone cannot be used to definitively identify the Pt adsorption site [32] , and a combined analysis approach of HAADF-STEM, XPS, XANES, and EXAFS must be used to corroborate the theory predicted representative structure, as these characterization results together set the context of platinum species size, chemical valence, and coordination environment. Identification of oxygen migration reaction mechanism To understand how the Pt 1 /CeO 2 and Pt-O-Pt/CeO 2 catalysts catalyze CO oxidation so differently, DFT calculations combined with mean-field microkinetic simulations were conducted to study the CO oxidation mechanism (the partial pressure for CO and O 2 are 0.001 and 0.05 bar, respectively, consistent with our reaction studies). The schemes for the CO oxidation cycles and geometric and energetic information are shown in Fig. 3 , Supplementary Figs. 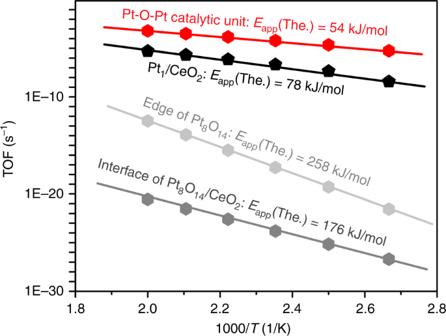Fig. 4 Microkinetic simulations for various CO oxidation routes on the Pt1/CeO2and Pt8O14/CeO2structures. The predicted apparent activation barriers,Eapp(The., theory predicted), are indicated 32 , 33 , and Supplementary Table 4 . 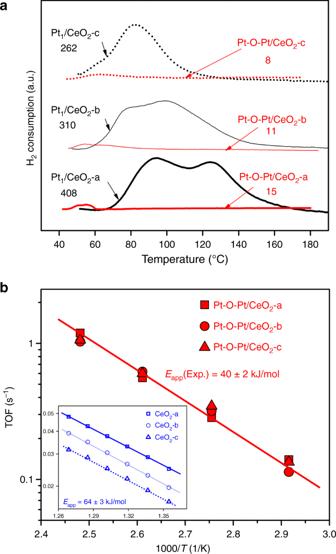Fig. 5 Catalyst surface [O] reducibility and site-specific turnover frequencies (TOFs) for CO oxidation reaction.aH2temperature programmed reduction (TPR) profiles and integrated amounts of reducible [O] for the Pt1/CeO2and Pt-O-Pt/CeO2catalysts. The labeled values inaare the integrated amount of reducible oxygen with the default unit of “µmol [O]/gcat.”bIdentical TOFs were found for the Pt-O-Pt/CeO2catalysts and different TOFs were found for the Pt-free ceria supports (inset) 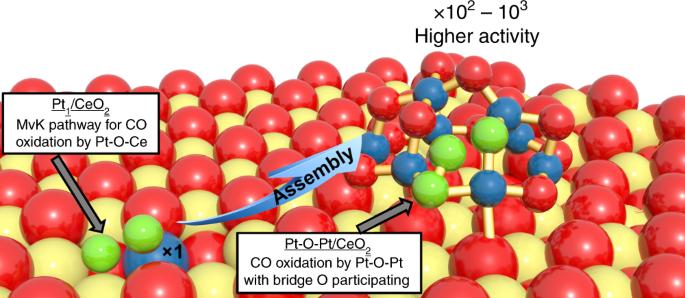Fig. 6 Different transition states for oxygen activation by the Pt1-O-Ce and the Pt-O-Pt ensembles. The detailed configurations for the CO oxidation cycles of the two groups of catalysts are illustrated in Fig.3. The Pt1single atoms are assembled into the more active Pt-O-Pt ensembles during the activation protocol. Color legend of atoms: Ce = yellow; Pt = blue; O = red; O atoms in the transition states for O2activation are green. MvK = Mars–van Krevelen On Pt 1 /CeO 2 (111) and Pt 8 O 14 /CeO 2 (111), the preferred pathway involves adsorbed CO on the Pt site during the CO oxidation cycle due to stronger adsorption of CO compared with O 2 at the same Pt site (Supplementary Table 5 ). CO oxidation is predicted to follow the Mars–van Krevelen (MvK) mechanism [33] , [34] , [35] at the square-planar Pt 1 -O 4 unit in Pt 1 /CeO 2 (Fig. 3a and Supplementary Table 4 ), where adsorbed CO on the Pt atom (CO Pt ) reacts with surface lattice oxygen (O Ce ) in CeO 2 with a moderate activation barrier ( E a <105 kJ/mol). O 2 dissociation ( E a = 150 kJ/mol) will heal the oxygen vacancy sites to complete the catalytic cycle on Pt 1 /CeO 2 . Based on microkinetic simulations, the predicted apparent activation energy ( E app ) on Pt 1 /CeO 2 is 78 kJ/mol (Fig. 4 ), which is in close agreement (within typical DFT errors of ±15 kJ/mol) with the experimentally measured apparent activation energy of 86 ± 3 kJ/mol. Degree of rate control analysis shows that O 2 dissociation is the rate-determining step (RDS) for CO oxidation on Pt 1 /CeO 2 (Supplementary Figs. 34a , 35a ). Fig. 3 Potential energy diagrams and configurations for CO oxidation cycle. CO oxidation proceeds on a the Pt 1 /CeO 2 and b at the Pt-O-Pt catalytic unit in Pt 8 O 14 /CeO 2 . CO adsorption energies and reaction barriers are indicated in kJ/mol in the potential energy diagram. The bond distance between the two fragments at the transition state (TS) is given in angstrom (Å) in the configurations of CO oxidation. Beige, red, and blue spheres are Ce, O, and Pt atoms, respectively. The small gray and green spheres are C and O atoms involved in CO oxidation. Corresponding energetics are given in Supplementary Table 4 Full size image Fig. 4 Microkinetic simulations for various CO oxidation routes on the Pt 1 /CeO 2 and Pt 8 O 14 /CeO 2 structures. The predicted apparent activation barriers, E app (The., theory predicted), are indicated Full size image For the Pt-O-Pt/CeO 2 samples, we have considered three potential catalytic cycles in the Pt 8 O 14 /CeO 2 system, namely: (1) at the platinum–ceria interface of Pt 8 O 14 /CeO 2 , (2) at the edge of Pt 8 O 14 , and (3) at the Pt-O-Pt site in Pt 8 O 14 . The first step for CO oxidation in scenario 1 is the removal of one oxygen atom in Pt 8 O 14 by CO Pt with an activation barrier of 26 kJ/mol (Supplementary Fig. 32 and Supplementary Table 4 ). Afterwards, CO oxidation may take place at the interface of Pt 8 O 14 /CeO 2 , obeying the MvK mechanism and involving O Ce removal and O 2 dissociation. The reaction of CO Pt with O Ce to form CO 2 has the highest activation barrier for CO oxidation ( E a = 151 kJ/mol), followed by O 2 dissociation ( E a = 72 kJ/mol). The predicted apparent activation energy is 176 kJ/mol at the metal–support interface of Pt 8 O 14 /CeO 2 , which results in a much too low CO oxidation rate compared with the experimental measurements (Fig. 4 ). The lower activity of the Pt 8 O 14 /CeO 2 interface compared with Pt 1 /CeO 2 originates from the weak CO adsorption on Pt 8 O 14 /CeO 2 ( E CO = −27 kJ/mol), resulting in low CO coverage (Supplementary Figs. 34b and 35b ). Although the platinum–ceria interface is accepted as the catalytic center for CO oxidation catalyzed by either single-atom Pt 1 /CeO 2 catalysts or classic nanoparticles/clusters supported on ceria [36] , [37] , the active site at the interface of our Pt 8 O 14 /CeO 2 system cannot rationalize the observed high activity of the Pt-O-Pt/CeO 2 catalysts under these oxygen-rich conditions at low temperatures. Alternatively, we probed the possible reaction route where CO oxidation proceeds solely on the Pt 8 O 14 and the CeO 2 support is a spectator (scenarios 2 and 3). At the Pt 8 O 14 edge atoms, O 2 physisorbs ( \(E_{{\mathrm{O}}_{2}}\) = −1 kJ/mol) after CO adsorption (Supplementary Fig. 33 and Supplementary Table 4 ). The RDS for CO oxidation is CO Pt + O 2 → CO 2 + O Pt with an activation barrier of 117 kJ/mol (Supplementary Figs. 34c , 35c and Supplementary Table 4 ). Consequently, the CO oxidation rate is still too slow at the Pt 8 O 14 edge atoms with an apparent activation energy of 258 kJ/mol (Fig. 4 ) due to the weak adsorption of O 2 and high barrier for CO Pt reacting with O 2 . Surprisingly, this work finds that the Pt-O-Pt ensemble in the Pt 8 O 14 (scenario 3) can facilitate an O migration mechanism to rapidly catalyze CO oxidation (Fig. 3b and Supplementary Table 4 ). One O atom from the adsorbed O 2 can migrate to a neighboring O atom in the Pt 8 O 14 to form O 2 v with an E a = 103 kJ/mol, followed by O Pt removal and O 2 v dissociation. The activation barriers for the O Pt atom reacting with CO Pt and O 2 v dissociation are predicted to be at least 26 kJ/mol lower than the O atom migration step; thus, O migration is the RDS for this mechanism (Supplementary Figs. 34d , 35d and Supplementary Table 4 ). The microkinetic simulations predict E app for the Pt-O-Pt/CeO 2 catalysts of 54 kJ/mol, which is close to our experimentally measured result of 40 ± 2 kJ/mol (Fig. 4 ). To probe the impact of other minor CeO 2 morphologies observed in experimental work (Supplementary Figs. 17 and 18 ) on the activity of Pt 8 O 14 , the rate-determining CO oxidation reaction step involving CO reacting with lattice oxygen is studied on Pt 8 O 14 /CeO 2 (110) and Pt 8 O 14 /CeO 2 (100). The representative Pt 8 O 14 structure on CeO 2 (111) surface searched by GCMC simulations is deposited on (110) and (100) facets with each Pt atom binding four oxygen atoms according to our XPS and EXAFS data. DFT calculations (Supplementary Fig. 36 ) show that CO oxidation at the interface of Pt 8 O 14 /CeO 2 (110) and Pt 8 O 14 /CeO 2 (100) is unfeasible due to a prohibitively high CO oxidation reaction barrier. Therefore, our analyses of platinum species on each of the common ceria surface facets allow us to infer that CO oxidation preferentially occurs on Pt-O-Pt ensemble rather than at the interface of Pt 8 O 14 /CeO 2 for (111), (110), and (100) facets. The measured reaction orders with respect to CO and O 2 are −0.2 and 0.4, respectively, for Pt 1 /CeO 2 , and 0.3 and ~0, respectively, for Pt-O-Pt/CeO 2 . These reaction orders corroborate the proposed reaction mechanism (see detailed derivation for reaction orders in Supplementary discussion below Supplementary Fig. 37 ). The indirect catalytic role of ceria predicted in this proposed catalytic route corroborates our experimental findings. As shown by the H 2 temperature programmed reduction (TPR) results (Fig. 5a ) of the reaction-spent catalysts, the more abundant reducible oxygen species from the platinum–ceria interface in the Pt 1 /CeO 2 catalysts did not count towards the superior catalytic performance of the Pt-O-Pt/CeO 2 catalysts. The ceria supports are essentially identical for the Pt 1 and Pt-O-Pt groups of reaction-spent catalysts according to Ce3 d and O1 s XPS spectra (Supplementary Fig. 4 ). Without the presence of the supported platinum, the [O] reduction in the ceria lattice by H 2 will not take place until above 200 °C (Supplementary Fig. 9b ). We attribute the major peak in the temperature range of 60–100 °C to the immediate [O] depletion at the six nearest oxygen atoms in the Pt 1 -O-Ce unit. The next H 2 consumption peak in the temperature range of 100–160 °C is related to the further depletion of the ceria lattice oxygen that can migrate to the Pt 1 -CeO 2 interfaces. In contrast, the Pt-O-Pt/CeO 2 catalysts do not display active [O] supply from the ceria to initiate the low-temperature oxidation. A trace amount of [O] reduction takes place in the temperature range of 40–60 °C for all three Pt-O-Pt/CeO 2 catalysts. To examine the impact of the ceria supports, the three types of ceria, a, b, and c, were first probed with the CO oxidation reaction as bare supports. The calculated TOFs per Ce site are quite different among the Pt-free ceria materials (Fig. 5b , inset), as they have different capacities in releasing atomic oxygen species to oxidize gas molecules such as H 2 and CO (Supplementary Figs. 9 and 10 ). In contrast, the same TOFs can be obtained when we calculate the TOFs per Pt atom from the various Pt-O-Pt/CeO 2 catalysts (Fig. 5b ). This finding shows that the highly active Pt-O-Pt catalytic unit overrides the influence of the different oxygen-supply capabilities from ceria in catalyzing the low-temperature CO oxidation reaction, and the uniformity of the catalytic units created by our activation procedure is remarkable. Fig. 5 Catalyst surface [O] reducibility and site-specific turnover frequencies (TOFs) for CO oxidation reaction. a H 2 temperature programmed reduction (TPR) profiles and integrated amounts of reducible [O] for the Pt 1 /CeO 2 and Pt-O-Pt/CeO 2 catalysts. The labeled values in a are the integrated amount of reducible oxygen with the default unit of “µmol [O]/g cat .” b Identical TOFs were found for the Pt-O-Pt/CeO 2 catalysts and different TOFs were found for the Pt-free ceria supports (inset) Full size image We also probed the possibility of creating similar Pt-O-Pt sites on an alumina support, in which the parent catalyst is the single-atom Pt 1 /La-Al 2 O 3 with a platinum loading of ~0.5 wt.% that we recently reported [11] . Through a similar redox activation protocol that we have applied to the Pt 1 /CeO 2 catalysts, we created an activated Pt/La-Al 2 O 3 catalyst having a portion of its platinum as the active Pt-O-Pt catalytic sites, according to CO-DRIFTS studies (Supplementary Fig. 38 ) and kinetic measurements of E app (41 ± 2 kJ/mol, Supplementary Fig. 39 ) and reaction orders (0.3 and 0.1 for CO and O 2 , respectively, Supplementary Fig. 37 ). This evidence further supports our hypothesis about the indirect role of the ceria particles (10–30 nm) in influencing the intrinsic low-temperature CO oxidation catalysis of Pt-O-Pt/CeO 2 under oxygen-rich conditions. It is worth noting that the concept of “maximized atom efficiency” is different from “maximized activity per atom.” Our results highlight that Pt 1 indeed has maximized its material utilization efficiency, but there is large room to improve the activity per Pt atom. The solution from this work is to tackle the issue of lacking neighboring Pt atoms in the typical Pt 1 /CeO 2 system. By forming the Pt-O-Pt catalytic unit in representative one-layer Pt 8 O 14 cluster, the Pt atoms can now effectively activate and utilize the oxygen intermediates to catalyze the low-temperature CO oxidation. A recent work adjusted the Pt-O coordination number between 2 and 3 in PtO x clusters by either reductive or oxidative treatment at 350 °C to modify the catalytic activity of PtO x /CeO 2 nanowire catalysts within one order of magnitude for the CO oxidation under oxygen-rich conditions [24] . Despite that the platinum was not fully exposed in this prior work, as the dispersion ranged from 10 to 83% (Supplementary Table 1 ), the authors may have created a portion of similar sites as we did in this work (best-performing catalysts from the current work are on average six times more active by incorporating the possible impact of different reactant concentrations). Here, by maintaining 100% platinum dispersion, which means that all the Pt atoms are accountable for surface catalysis and there is a minimal amount of spectator Pt species to distort the averaged characterization results, we found that the coordination number of Pt-O may not be the most decisive factor for the much more dramatic change of the CO oxidation activity, because both our Pt 1 and Pt-O-Pt structures have four oxygen atoms directly bonded to the platinum center at the starting point of each catalytic cycle. More importantly, the synergistic effect of the two, paired, platinum atoms in the Pt-O-Pt ensemble provides an alternative oxygen supply route independent of ceria substrates. This intrinsic catalytic difference between the isolated Pt 1 and the paired Pt-O-Pt structure could likely not be overcome by merely changing the Pt-O coordination numbers and considering each Pt atom as an independent unit. The mechanistic importance of the Pt-O-Pt interaction is highlighted in this work, where most of the attention was on the Pt-O-Ce interaction in previous studies. As shown in Fig. 6 , the rate-determining steps of the CO oxidation reaction by Pt 1 /CeO 2 and Pt-O-Pt/CeO 2 catalysts involve different sites and mechanisms for oxygen activation. The CO oxidation reaction proceeds through the MvK mechanism at the Pt 1 -O-Ce interface in the Pt 1 /CeO 2 catalyst, while the reaction is more efficiently catalyzed by the Pt-O-Pt/CeO 2 catalyst at its Pt-O-Pt unit with the bridge -O- participating. The similar feature might be shared with other oxide clusters having high metal dispersion and abundant undercoordinated metal sites. Fig. 6 Different transition states for oxygen activation by the Pt 1 -O-Ce and the Pt-O-Pt ensembles. The detailed configurations for the CO oxidation cycles of the two groups of catalysts are illustrated in Fig. 3 . The Pt 1 single atoms are assembled into the more active Pt-O-Pt ensembles during the activation protocol. Color legend of atoms: Ce = yellow; Pt = blue; O = red; O atoms in the transition states for O 2 activation are green. MvK = Mars–van Krevelen Full size image The findings from this work should only be cautiously extended to a general type of clusters that retain a layered three-dimensional structure, where the lower dispersion and more saturated coordination environment of platinum bring more uncertainties. However, we infer that the Pt-O-Pt catalytic unit defined in this work is a prototype that illustrates an important advantage of catalysts with neighboring metal centers for efficient oxygen activation. Several recent reports are now indicating a general sense of agreement about the concept of using PGMs to create PGM-O-PGM catalytic units. Recent work by Zhao et al. [38] report a synthesis of a Ir-O-Ir structure on α-Fe 2 O 3 , and the synergistic effects between the two nearby iridium atoms were inferred to explain the 2.6 times higher activity of the dinuclear structure from its single-Ir atom counterpart for solar water oxidation. Jeong et al. [39] reported that the Rh 1 /CeO 2 catalyst has low activity for C 3 H 6 and C 3 H 8 oxidation, but another speculated Rh ensemble catalyst is highly active for C 3 H 6 and C 3 H 8 oxidation. The elusive Rh ensembles cannot be observed in HAADF-STEM images, and the k 3 -weighted EXAFS radial distribution indicates two sets of Rh-O-Rh bonds with coordination numbers near 0.6 (means not even a dinuclear structure—instrumental signal limitations). More recently, Dessal et al. [40] confirmed an enhancement of CO oxidation activity of the Pt/γ-Al 2 O 3 catalysts when the Pt 1 atoms were agglomerated into platinum oxide clusters with a Gaussian distribution of cluster sizes from 0.5 to 1.5 nm. These studies are using different PGM species, supports, PGM domain sizes, and different reactions, but the formation of the paired PGM-O-PGM bond is the common variable behind the improved catalytic performance. We believe this is where the general implication of this material development and mechanistic investigation work resides. One should also avoid oversimplifying this work as any dinuclear Pt-O-Pt structures can be more active than the single-atom Pt species in activating [O] intermediates. Notably, one of the platinum atoms in this highly active Pt-O-Pt catalytic unit does not have any direct -O- linkages to the ceria support, and it is in fact the enabler for facile O migration and fast CO oxidation. Indeed, the lattice oxygen of ceria is critical for the formation of stable Pt-O bonds according to our XAS analyses. However, the ceria is also shown to be largely a spectator species in the low-temperature CO oxidation reaction catalyzed by the Pt-O-Pt/CeO 2 systems. We envision that, if the Pt-O-Pt unit can be stabilized through similar oxygen linkages, a similar catalytic species may be created on various support substrates other than ceria. The formation of a Pt-O-Pt structure on activated Pt/La-Al 2 O 3 supports this hypothesis (Supplementary Figs. 37 – 39 ), but developing alternative preparation methods to build the exclusive catalytic sites on the alumina support needs further effort that is outside the scope of this work. The exception from the general assessment of the present work is most likely to happen when quantum-size effects become evident in small ceria nanoclusters (especially <5 nm). Elegant studies showed that the oxygen vacancy formation in CeO 2 nanoclusters exposing small O-terminated (111) and (100) facets is more probable compared to the extended CeO 2 surfaces [41] , [42] , [43] , [44] . Theoretical evidence shows that the oxygen reverse spillover from these small ceria nanoparticles to the supported Pt species can generally be a more favorable process compared with Pt species supported on larger ceria particles, the latter of which is typically represented by slab computational models [9] , [45] , [46] . Such an unusually high oxygen mobility from the ceria have been predicted by modeling studies on CeO 2 nanoclusters comprising from about 60 to over 200 atoms, where the largest Ce 140 O 180 has an approximate size of ~2.4 nm [42] , [47] , [48] . The supporting experimental evidence was provided by carefully growing small Pt/CeO 2 nanoparticles on a CeO 2 (111) film under ultrahigh vacuum—these grown ceria nanoclusters are only about ~3 nm in diameter and 0.4 nm in height [29] , [43] . We emphasize that the these CeO 2 nanoclusters (up to ~3–4 nm) with extraordinary capability for generating mobile oxygen species are intrinsically different from the 10–30 nm ceria particles (homemade and commercial) used in this work. For example, small ceria nanoparticles of 3–4 nm were shown to improve the catalytic activity of gold species for CO oxidation by about two magnitudes [49] , [50] , but this highly active oxygen supply disappears quickly for regular ceria nanoparticles that are larger than 10 nm in automotive applications [51] , [52] , [53] . Typical calcination treatment from 300 to 800 °C to fully decompose cerium precursors and to form stable ceria structures usually leads to the CeO 2 particle size from 10 to 30 nm [51] , [52] . These ceria particles have abundant stable CeO 2 (111) facets [54] , [55] . These differences lead to the observation that our single-atom Pt 1 (IV)-O 4 is mostly observed on the stable CeO 2 (111) surfaces of a 10–30 nm ceria particle, although a sinter-resistant single-atom structure Pt 1 (II)-O 4 sits at the less stable CeO 2 (100) nanofacets of the small ceria nanoclusters (e.g., 1–3 nm) [29] , [56] . Of course, the small fraction of rounded edges, steps and kinks in our 10–30 nm ceria particles may well have led to the presence of a tiny portion of active sites as Pt-O-Pt plus active ceria substrates. These nonuniformities could be part of the reason for the deviations of kinetics between the computational results and experimental measurements. A success of synthesizing and stabilizing tiny ceria nanoclusters and anchoring an appreciable amount of the targeted platinum structure (e.g., the Pt-O-Pt) onto them bodes the ultimate solution of best using both the platinum and ceria substrate. However, the bottom line is, when widely available ceria particles with larger size (>10 nm) and mediocre oxygen mobility are being adopted as an industrial catalyst support, activating the single-atom Pt to form the paired Pt-O-Pt ensemble is an effective way to create an alternative oxidative reaction pathway to benefit the low-temperature reactions. These tunable catalytic systems, either at a single-atom form or a Pt-O-Pt structure, may serve as powerful platforms for future studies of many other reactions. Catalyst preparation Platinum was loaded onto the ceria supports by a strong electrostatic adsorption method [57] . H 2 PtCl 6 was chosen as the platinum precursor, because the platinum–ligands complex anions can evenly adsorb on the positively charged –O-Ce-OH 2 + surface sites on ceria as single-atom layers when the pH of the solution is below the point of zero charge of ceria. To begin, the pH value of the H 2 PtCl 6 solution was adjusted to pH ≈ 9 by ammonia. The transparent solution was stirred at 70 °C overnight to allow the substitution of -Cl in [PtCl 6 ] 2− by -OH in solution. The as-prepared ceria powder was then added into the solution to adsorb the preformed [Pt(OH) 6 ] 2− as a single-atom Pt layer. The concentrations of the platinum precursor and the amount of ceria were varied to keep the same solid–liquid contact interface of 500 m 2 /L. We washed the filtration cake (filtered catalyst) with a total of 2 L distilled water at 80 °C during each sample filtration. The obtained samples were dried at 100 °C overnight, then calcined in air at 500 °C for 3 h, followed by H 2 reduction at 250 °C for 0.5 h to further remove any possible residual -Cl, and finally calcined in air at 500 °C for 1 h. These Pt 1 /CeO 2 samples are hereafter referred to as the “as-prepared” catalysts, and designated as “Pt 1 /CeO 2 -a, Pt 1 /CeO 2 -b, and Pt 1 /CeO 2 -c”. None of the Pt-containing components were detected as crystallized structures (Supplementary Figs. 6 – 8 , 11 – 16 ), and limited changes happened to the BET surface areas, that is, they changed to 74, 60, and 44 m 2 /g from 80, 64, and 51 m 2 /g, respectively. Our Pt 1 /CeO 2 samples were calcined at 500 °C, so the bulk diffusion of the Pt into CeO 2 that usually occurs above 700 °C is limited [58] , [59] . The nearly 100% Pt dispersion (measured at room temperature by a CO chemisorption method that passivates the ceria support in directly contributing to CO adsorption [39] , [60] , [61] ) and the measured catalytic activity in line with published data (Supplementary Table 1 ) confirm that the Pt 1 species are accessible to the reactants. After mild reduction at 200 °C in 5% H 2 , and subsequent exposure of these Pt 1 /CeO 2 catalysts to a CO plus O 2 feed stream ([CO] = 1000 ppm, [O 2 ] = 5%, balanced with N 2 ) at ambient temperature, we saw a notable enhancement of catalytic activity due to the restructuring of the platinum species. The reason for using diluted H 2 at mild temperatures is to adequately break the Pt-O bond that holds the single-atom Pt in place while avoiding extensive metal Pt sintering [30] , [31] , [62] . Our optimizations for reduction temperature and time are shown in Supplementary Fig. 1 . Here, mild H 2 reduction at 200 °C breaks the Pt-O-Ce bond in the Pt 1 -O x single-atom structure, because all the reducible oxygen species near Pt–ceria interface are consumed below 200 °C according to H 2 -TPR for the Pt 1 /CeO 2 catalysts (Fig. 5a ). During the optimized H 2 reduction phase, we expect the single-atom Pt 1 /CeO 2 catalysts to generate abundant undercoordinated Pt atoms as nanorafts under the rather mild reduction condition and relatively short reduction time [30] , [31] , [62] . During the phase of reoxidation using a mixture of CO plus O 2 , both CO and O 2 can induce a Pt restructuring depending on their respective pressure [63] , [64] , [65] , [66] . In general, O 2 molecules tend to coordinate with Pt to form nano islands of multilayered α-PtO 2 -like oxides [67] . This is an unwanted outcome for the scope of this work, because the formation of the multi-layer spherical platinum oxide structures may result in the creation of Pt atoms with nonuniform chemical environment depending on their relative location in the platinum particle and from the ceria support. Characterizing such a mixed batch of catalytic species will generate average quantities and even distorted results, which will mask the characteristics of the active species [4] , [6] . Some Pt atoms may also be buried in the particle bulk, losing their ability to catalyze surface reactions. To prevent the formation of bulk particles, CO molecules were added to attach to Pt surfaces as ligands to cause CO-CO repulsion between nearby Pt sites [65] . As shown in Supplementary Fig. 2 , having a trace amount of CO in the diluted oxygen feed stream is indeed helpful to activate the catalysts. These treatment steps lead to the formation of the Pt-O-Pt structure on ceria according to our characterization studies. Therefore, these activated samples are denoted as “Pt-O-Pt/CeO 2 .” We excluded the impact of chloride on the change of catalytic activities, as all our Pt 1 /CeO 2 and Pt-O-Pt/CeO 2 catalysts show a minimal and similar chloride concentration of 70–90 ppm according to ion chromatography analysis. The Pt-related catalytic sites were characterized by STEM, CO chemisorption, XPS, XAS, and H 2 TPR after exposure to reaction conditions as the working catalysts. CO oxidation tests and kinetics The CO oxidation reaction was conducted in a packed-bed tubular reactor. A 25 mg powder sample was diluted with 200 mg quartz sand in the catalyst bed. The catalysts were tested in an O 2 -rich gas atmosphere to reflect the lean-burn gasoline and diesel engine conditions. The test procedures were as follows: first, we ramped up the reactor temperature to 500 °C in 20% O 2 balanced with N 2 at a heating rate of 10 °C/min, and held for 30 min. Next, we cooled down the reactor to near-ambient temperature with an N 2 purge until the temperature of the catalyst bed was stable. After the CO oxidation reaction feed stream ([CO] = 1000 ppm, [O 2 ] = 5%, balanced with N 2 at a flow rate of 1000 mL/min) was switched in. The steady-state and light-off conversion rates were measured at elevated temperatures after the baseline readings became stable at near-ambient temperature. To activate the as-prepared sample, a treatment including a reduction at 200 °C in 5% H 2 for 15 min and a subsequent exposure to the CO plus O 2 atmosphere at ambient temperature was used before the reaction. Wet CO oxidation followed the same test procedure with a feed stream containing 3% H 2 O ([CO] = 1000 ppm, [O 2 ] = 5%, [H 2 O] = 3%, balanced with N 2 at a flow rate of 1000 mL/min). The concentrations of CO and CO 2 were monitored by an MKS 2030 gas cell Fourier-transform infrared spectroscopy, and the O 2 concentration was measured by mass spectroscopy (Hiden HPR20). Kinetic measurements were carried out on the same equipment setups. A typical flow rate ranging from 1200 to 1500 mL/min was used for 10 to 20 mg of catalyst in each test to ensure the catalytic reaction was free of heat and mass transfer effects. The CO conversion was therefore kept below 20% for all the reaction rate measurements. DFT modeling approach Spin-polarized DFT calculations were performed using the Vienna Ab initio Simulation Package (VASP) [68] , [69] with the projector augmented-wave method to treat electron–ion interactions [70] . The Perdew–Burke–Ernzerhof (PBE) exchange-correlation functional [71] was used as the density functional approximation for all genetic algorithm (GA) and GCMC calculations. The revised Perdew–Burke–Ernzerhof (RPBE) exchange-correlation functional [72] was used to calculate the CO oxidation catalytic cycle because of its superior ability to predict accurate adsorption energies over PBE as compared with the experiment [72] . The strongly correlated 4 f electron of cerium was treated with the DFT + U correction, using a U eff = 5 eV for both PBE and RPBE calculations [73] . Brillouin zone sampling was restricted to the Γ point for all DFT calculations. To avoid artificial self-interactions between slabs due to periodic boundary conditions, the surface slabs were separated by a vacuum layer of 15 Å. A GA was used to find the global minimum structure of a Pt 8 cluster supported on ceria (Pt 8 /CeO 2 ). The most stable Pt 8 /CeO 2 structure is used as the initial configuration for the GCMC simulations. For the GA and GCMC simulations, a p (4 × 4) CeO 2 (111) surface with one O-Ce-O layer was used as the support model without geometry relaxation to improve the calculation efficiency. We did not include the presence of persistent oxygen vacancies on CeO 2 (111) surfaces during our CO oxidation mechanistic studies, as their rapid healing has been demonstrated by both theory and experiments [16] , [17] , [18] , especially under oxygen-rich reaction conditions [17] . The plane-wave cutoff energy was set to 300 eV and the convergence threshold for geometry optimizations was specified to 10 –3 eV for both GA and GCMC calculations. A p (4 × 4) CeO 2 (111) surface with two O-Ce-O layers was used as the support for studying the CO oxidation catalytic cycle on both the Pt 1 /CeO 2 (111) and Pt 8 O 14 /CeO 2 (111) systems. To analyze the impact of the exposed ceria facet on CO oxidation, the representative Pt 8 O 14 structure searched by GCMC [18] simulations on CeO 2 (111) was deposited on two O-Ce-O-layered (110) and (100) surfaces with each Pt atom binding four oxygen atoms according to our XPS and EXAFS data. Experimental observations [74] , [75] suggest that the (100) surface is terminated by 0.5 monolayer of oxygen. To obtain a consistent model, we constructed the oxygen terminated (100) surface by removing half of the oxygen atoms on the top and bottom surfaces (Supplementary Fig. 36 ). The top O-Ce-O layer, adsorbates, Pt single atom, and Pt 8 O 14 cluster could relax during geometry optimization and transition state searches. A plane-wave basis with a cutoff energy of 400 eV was chosen. The climbing-image nudged elastic band (CI-NEB) method [76] , [77] was used to find the transition states involved in the CO oxidation mechanism. The CI-NEB force tolerance was set to 0.05 eV/Å. CO vibrational frequency was calculated within the harmonic approximation. The calculated vibrational frequency of gaseous CO by DFT-RPBE was 2105 cm −1 , which is 65 cm −1 smaller than the true value measured in our experiment (2170 cm −1 ). Thus, we applied a 65 cm −1 rigid shift to all the calculated CO vibrational frequencies on Pt 1 /CeO 2 and Pt 8 O 14 /CeO 2 catalysts to compare with our experimental DRIFTS spectra. The zero-point energy correction was not considered. Details on GA and GCMC simulations as well as the mean-field microkinetic simulations approach are presented in the Supplementary Information .